RETRACTED ARTICLE: Reduction of carbon dioxide to oxalate by a binuclear copper complex Reduction of carbon dioxide to products such as oxalate (C 2 O 4 2− ) is an active area of research, as the process converts an environmental pollutant into more useful organic compounds. However, carbon dioxide reduction remains a major challenge. Here we demonstrate a three-step reaction sequence in which a copper complex converts carbon dioxide to oxalate under mild conditions. The copper(II) complex is reduced to copper(I) in solution, either electrochemically or using sodium ascorbate. The reduced complex selectively reacts with carbon dioxide from air and fixes it into oxalate, with the oxalate ion bridging between two copper atoms. The bound oxalate ion is released as oxalic acid on treatment with mineral acids, regenerating the original copper(II) complex. This completes the process for conversion of carbon dioxide into oxalate using a binuclear copper complex and a mild reducing agent. Conversion of carbon dioxide to value-added organics has been an active area of research due to the likely role of CO 2 in global climate change as well as depletion of fossil fuel resources. Although CO 2 is a cheap, non-toxic and abundant potential carbon feedstock [1] , it is difficult to reduce to more useful forms due to its thermodynamic stability and kinetic inertness. Approaches to activating and reducing CO 2 by electrochemical and electrocatalytic methods in the presence of transition metals and their alloys have been reviewed extensively [2] , [3] , [4] , [5] , [6] , [7] , [8] , [9] , [10] . An attractive scheme for CO 2 reduction should be able to function under the mildest possible reaction conditions. There have been several reports of reduction of CO 2 to oxalate by low-valent d-block [11] , [12] , [13] , [14] , [15] and f-block metal complexes [16] , [17] , [18] . The Limberg group recently used β-diketiminate-based nickel(I) complexes to reduce CO 2 to CO or C 2 O 4 2− in multi-step processes [19] . One limitation of their system is the requirement of an extremely powerful reducing agent, KC 8 , to reduce Ni(II) to Ni(I). Bouwman and co-workers reported a binuclear copper(I) complex that can reduce carbon dioxide to oxalate, forming a tetranuclear copper(II) oxalate complex. They released oxalate by electrolysis in the presence of lithium perchlorate as supporting electrolyte to complete an electrocatalytic cycle [20] . Instead of using two molecules of binuclear Cu(I) complex for reductive coupling of CO 2 molecules as depicted in Bouwman’s work, we wished to prepare a single macrocyclic complex that can serve as a host for CO 2 reduction. We chose the m -xylylene group as a spacer to connect our two pyridyltriazole chelating units [21] . Other researchers have used multifunctional ligands to control the spatial position of two metal centres. Some of the best known examples are the cofacial diporphyrins, which are capable of catalyzing multielectron redox processes [22] , [23] , [24] . Several research groups have prepared complexes from dipyridyltriazoles (though they lead to relatively short metal–metal distances) [25] ; other binucleating ligands have also been employed [26] . We report herein a binuclear metallacyclic copper complex that can selectively capture CO 2 from air and reduce it to oxalate, in the form of an oxalate-bridged complex. The oxalate-bridged complex releases oxalic acid when it is treated with dilute mineral acid, regenerating the original copper complex. Synthesis of binuclear copper(II) complexes The complexation of m -xpt with CuX 2 (X=NO 3 , Cl) gave dimeric macrocycles, [Cu 2 ( m -xpt) 2 (NO 3 ) 2 ](NO 3 ) 2 and [Cu 2 ( m -xpt) 2 Cl 2 ]Cl 2 (ref. 21 ). Although the distance between the two Cu centres in these compounds is appropriate for small-molecule guests, they are insoluble in common organic solvents. To improve their solubility and hence widen the scope of host–guest chemistry, we replaced the anions with the more hydrophobic PF 6 − ( Fig. 1 ): metathesis gave [Cu 2 ( m -xpt) 2 (NO 3 ) 2 ](PF 6 ) 2 , 1 , and [Cu 2 ( m -xpt) 2 Cl 2 ](PF 6 ) 2 , 2 (see crystal structures in Supplementary Figs. 1 and 2 ), respectively. 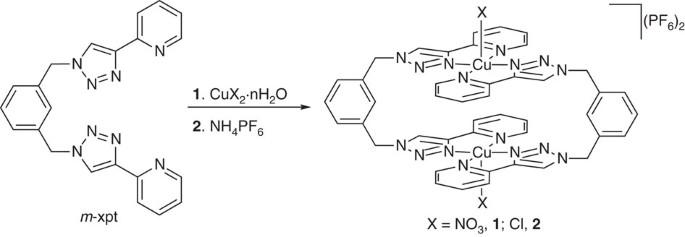Figure 1: Synthesis of complexes 1 and 2. Complexation of them-xpt ligand with Cu2+gives dimeric macrocycles that are water soluble, but become organic soluble when their counter anions are replaced with PF6−. Figure 1: Synthesis of complexes 1 and 2. Complexation of the m -xpt ligand with Cu 2+ gives dimeric macrocycles that are water soluble, but become organic soluble when their counter anions are replaced with PF 6 − . Full size image Reduction of Cu(II) complexes Cyclic voltammetry (CV) of 1 and 2 in dimethylformamide (DMF) showed quasi-reversible waves at ~0.28 V versus Ag/AgCl (−0.27 V for complex 1 and −0.28 V for complex 2 versus Fc/Fc + ; see Supplementary Fig. 3 and Supplementary Table 1 ). These results prompted us to investigate the reactivity of the Cu(I) dimers obtained by reducing complex 1 or 2 . For chemical reduction of Cu(II) to Cu(I), we used sodium ascorbate [27] , as is frequently done to produce Cu(I) catalysts in situ for the well-known ‘click’ (azide-alkyne cyclization) reaction [28] , [29] . As shown in Fig. 2 , treatment of 1 or 2 with sodium ascorbate in DMF under N 2 gave a yellow copper(I) complex. During this reaction, the Cu(II) d–d electronic absorption band disappears, and an intense new band at 384 nm appears ( Supplementary Figs. 4 and 5 ). We attribute the 384 nm ( ε =1.05 × 10 4 M −1 cm −1 ) band to a metal-to-ligand charge transfer transition in the macrocyclic Cu(I) complex [Cu 2 ( m -xpt) 2 ](PF 6 ) 2 , 3 . This new compound is stable in air for several days in the solid state. Although this was surprising at first, similar air stability of mononuclear Cu(I) pyridyltriazole complexes has been reported by Petitjean et al . 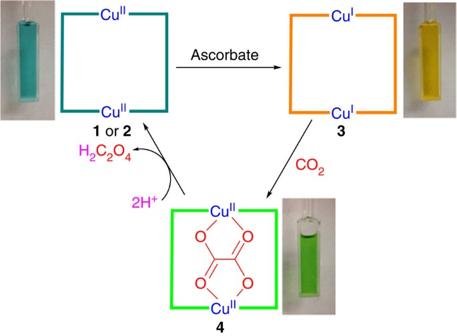Figure 2: Three-step reaction cycle for reduction of carbon dioxide. The starting copper(II) complexes (1and2) are reduced to Cu(I) complex3in the presence of sodium ascorbate. Complex3reacts with CO2to give oxalate-bridged complex4. The oxalate is released in the form of oxalic acid when complex4is treated with acids, regenerating the starting ‘empty’ complexes. [30] Figure 2: Three-step reaction cycle for reduction of carbon dioxide. The starting copper(II) complexes ( 1 and 2 ) are reduced to Cu(I) complex 3 in the presence of sodium ascorbate. Complex 3 reacts with CO 2 to give oxalate-bridged complex 4 . The oxalate is released in the form of oxalic acid when complex 4 is treated with acids, regenerating the starting ‘empty’ complexes. Full size image Reduction of CO 2 to oxalate by Cu(I) Solutions of 3 , generated in situ by reduction of 1 or 2 with sodium ascorbate in DMF, react with CO 2 (g) to produce the oxalate-bridged Cu(II) dimer [Cu 2 ( m -xpt) 2 ( μ -C 2 O 4 )](PF 6 ) 2 , 4 . The progress of the reaction was monitored by electronic absorption spectroscopy. We examined both the appearance of the Cu(II) d-d band in 4 ( λ max =751 nm, ε =98 M −1 cm −1 ; Fig. 3 ); and the disappearance of the Cu(I) MLCT band at 384 nm, under CO 2 maintained at 1 atm ( Supplementary Fig. 6 ). The reaction was nearly complete after 128 h. Under these conditions, the appearance of the oxalate complex follows pseudo-first-order kinetics, with a rate constant of ~0.019 h −1 . The Fourier-transform infrared (FTIR) spectrum of 4 shows ν CO =1670, cm −1 ; an analogous experiment with 13 CO 2 yields ν CO =1651, cm −1 ( Supplementary Fig. 7 ). 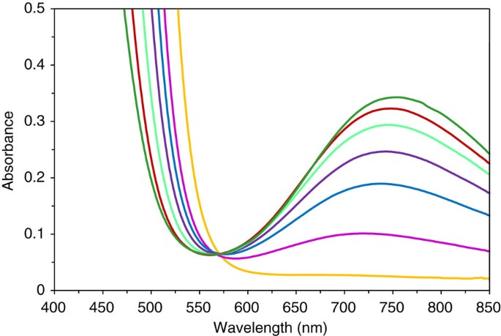Figure 3: Spectral changes during reduction of CO2to oxalate. A 3.76 mM solution of [Cu2(m-xpt)2](PF6)2,3, generatedin situfrom complex1in DMF using sodium ascorbate (1.5 equivalent), was kept under N2for 48 h (yellow), followed by oxidation by CO2. The remaining spectra, after 8 h (magenta) and then every 24 h to 128 h (dark green), demonstrate gradual formation of [Cu2(m-xpt)2(μ-C2O4)]2+,4(λmax=751 nm). Figure 3: Spectral changes during reduction of CO 2 to oxalate. A 3.76 mM solution of [Cu 2 ( m -xpt) 2 ](PF 6 ) 2 , 3 , generated in situ from complex 1 in DMF using sodium ascorbate (1.5 equivalent), was kept under N 2 for 48 h (yellow), followed by oxidation by CO 2 . The remaining spectra, after 8 h (magenta) and then every 24 h to 128 h (dark green), demonstrate gradual formation of [Cu 2 ( m -xpt) 2 ( μ -C 2 O 4 )] 2+ , 4 ( λ max =751 nm). Full size image The crystal structure of 4 ( Fig. 4 ) contains dimeric cationic complexes with crystallographically imposed 2/ m ( C 2h ) symmetry. The Cu···Cu separation (5.4213(7) Å), and the distances within the bridging oxalate ligand (C–C 1.544(7) Å; C–O 1.248(3) Å), are similar to those observed in other C 2 O 4 2− -bridged copper complexes [12] , [13] , [20] . 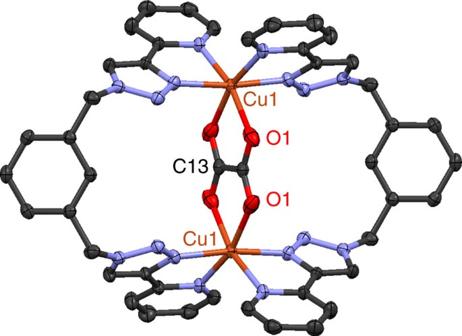Figure 4: Crystal structure of compound 4. In this complex, the oxalate ion in the centre has been formed by the reduction of CO2, and the two copper atoms are separated by 5.4213(7) Å. In this and other crystal-structure drawings, ellipsoids are at the 50% probability level, and hydrogen atoms, uncoordinated counter anions, and uncoordinated solvent molecules are omitted for clarity. Figure 4: Crystal structure of compound 4. In this complex, the oxalate ion in the centre has been formed by the reduction of CO 2 , and the two copper atoms are separated by 5.4213(7) Å. In this and other crystal-structure drawings, ellipsoids are at the 50% probability level, and hydrogen atoms, uncoordinated counter anions, and uncoordinated solvent molecules are omitted for clarity. Full size image We tested the selectivity of the reaction of complex 3 with CO 2 , by generating the Cu(I) dimer as described above and allowing the solution to evaporate in air in a petri dish or watch glass. After slow evaporation of the DMF we isolated complex 4 ( Supplementary Fig. 8 ) in high yield (96% from 1 ; 69% from 2 ). This conversion demonstrates selective reaction of [Cu 2 ( m -xpt) 2 ] 2+ , 3 , with CO 2 over O 2 . Removal of bound oxalate We also removed the coordinated oxalate from 4 , to regenerate the ‘empty’ Cu(II) macrocycle [Cu 2 ( m -xpt) 2 ] 4+ . Addition of HCl(aq) (8 eq) or HNO 3 (aq) (8 eq) to a suspension of complex 4 in methanol gave a green-blue solution, which deposited a green or blue-green precipitate over a period of 3 h. Crystallization from DMF–H 2 O gave the ‘empty’ host complexes [Cu 2 ( m -xpt) 2 Cl 2 ]Cl 2 [21] and [Cu 2 ( m -xpt) 2 (H 2 O) 2 ](NO 3 ) 4 , 5 ( Fig. 5 ), from the reaction of complex 4 with HCl and HNO 3 , respectively. The yields of empty complexes after HX treatment were nearly quantitative: 94% (HCl) and 96%(HNO 3 ). The oxalic acid produced in these reactions was characterized by 13 C nuclear magnetic resonance ( 13 C NMR; 163.2 ppm) and FTIR ( ν CO =1668, cm −1 ; with 13 CO 2 , 1642, cm −1 ) spectroscopy. 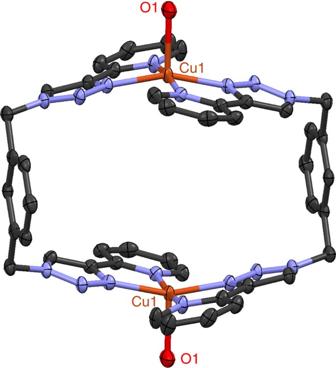Figure 5: Crystal structure of compound 5. The oxalate ion in compound4has been removed by treatment with nitric acid, liberating oxalic acid and leaving the ‘empty’ copper(II) complex [Cu2(m-xpt)2(H2O)2](NO3)4,5(Cu···Cu 7.2441(8) Å). This product is very similar to the starting complex1. Figure 5: Crystal structure of compound 5. The oxalate ion in compound 4 has been removed by treatment with nitric acid, liberating oxalic acid and leaving the ‘empty’ copper(II) complex [Cu 2 ( m -xpt) 2 (H 2 O) 2 ](NO 3 ) 4 , 5 (Cu···Cu 7.2441(8) Å). This product is very similar to the starting complex 1 . Full size image Oxalate as a guest As a complement to the above reaction, displacing bound oxalate from 4 , we also tested the ability of the empty copper(II) macrocycles to accept oxalate ion as a guest. Reaction of 1 and 2 with tetrabutylammonium oxalate [31] in acetonitrile yielded [Cu 2 ( m -xpt) 2 ( μ -C 2 O 4 )] 2+ , as confirmed by single crystal X-ray analysis. We have designed a metal-organic supramolecular system that reduces carbon dioxide to oxalate under mild reaction conditions. This binuclear Cu complex provides an unusual environment that promotes the binding and reduction of two CO 2 molecules. Although the fixation of CO 2 is slow, the Cu(I) dimer reacts selectively with CO 2 over O 2 . Oxalic acid is readily released from this product, regenerating the original ‘empty’ macrocycles. Cyclic voltammograms of 1 and 2 were unaffected by the addition of CO 2 (g). This is consistent with the low rate of reaction of [Cu 2 ( m -xpt) 2 ] 2+ ( 3 ) with CO 2 . Also, we observed no catalytic waves in CV experiments with 1 and 2 on addition of acid; thus, our complexes are not good electrocatalysts for H + reduction. We are currently experimenting with modified pyridyltriazole ligands to determine whether the complexes can be made more reactive with CO 2 , and developing alternate methods for the removal of oxalate; these changes are designed to develop the system into a catalytic cycle. General All commercially available reagents and solvents were purchased from Aldrich and Alfa Aesar and used without further purification. NMR spectra were recorded on a Bruker AV-400 MHz spectrometer. Electrospray ionization (ESI) mass spectra (MS) were measured on an Agilent 6210 instrument. FTIR spectra were recorded on a Bruker Tensor 27 spectrometer in attenuated total reflectance mode. Elemental analyses were performed by M-H-W Laboratories, Phoenix, Arizona. Ultraviolet-visible spectra were recorded on an Aviv 14DS spectrometer, with the samples in sealed combination flask-cuvettes. CV measurements were performed using a Princeton Applied Research Model 273A potentiostat/galvanostat with Power Suite 2.53 software. The measurements were carried out in DMF (0.1 M Bu 4 NPF 6 ), with glassy carbon working electrode, Ag/AgCl reference electrode, and Pt wire counter electrode. The ligand, m -xpt, was synthesized by using a literature procedure [21] . Preparation of [Cu 2 ( m -xpt) 2 (NO 3 ) 2 ](PF 6 ) 2 (1) To a stirred solution of Cu(NO 3 ) 2 ·3H 2 O (0.612 g, 2.54 mmol) in acetonitrile (75 ml), m -xpt (1.00 g, 2.54 mmol) in chloroform (50 ml) was added dropwise. The reaction mixture was allowed to stir at room temperature for 2 h. The precipitate was collected by filtration, washed with acetonitrile and chloroform, and dried to give a blue solid [Cu 2 ( m -xpt) 2 (NO 3 ) 2 ](NO 3 ) 2 (1.57 g, 1.35 mmol). The product was dissolved in water (200 ml), and an aqueous solution of NH 4 PF 6 (1.32 g, 8.09 mmol) was added. The mixture was stirred for 10 min and filtered. The precipitate was collected, washed with water, and dried in air to give 1 (1.84 g, 84%) as a light-blue powder. ESI-MS: m/z 1349.078, [Cu 2 ( m -xpt) 2 (PF 6 ) 3 ] + (calcd 1349.082). Microanalysis (Anal.). Calculated (Calcd) for [Cu 2 ( m -xpt) 2 (NO 3 )](PF 6 ) 3 ·H 2 O: C 36.93, H 2.68, N 16.64. Found: C 36.88, H 2.92, N 15.40. We found a consistently low percentage of nitrogen on microanalysis. This may be due to the presence of species such as [Cu 2 ( m -xpt) 2 ](PF 6 ) 4 in the product. However, when the product was crystallized by vapour diffusion of diethyl ether into its solution in DMF containing benzene, we isolated [Cu 2 ( m -xpt) 2 (NO 3 ) 2 ](PF 6 ) 2 ( Supplementary Fig. 1 and Supplementary Data 1 ). Preparation of [Cu 2 ( m -xpt) 2 Cl 2 ](PF 6 ) 2 (2) To a stirred solution of [Cu 2 ( m -xpt) 2 Cl 2 ]Cl 2 [21] (2.00 g, 1.86 mmol) in water (300 ml), excess NH 4 PF 6 (1.82 g, 11.2 mmol) was added. The mixture was stirred for 10 min. The precipitate was collected by filtration, washed with water, and dried to give 2 (2.05 g, 86%) as a blue-green solid. A crystalline product was obtained from DMF by vapour diffusion of diethyl ether ( Supplementary Fig. 2 and Supplementary Data 2 ). ESI-MS: 1239.085 [Cu 2 ( m -xpt) 2 (PF 6 ) 2 Cl] + (calcd 1239.087). Anal. Calcd for [Cu 2 ( m -xpt) 2 Cl 2 ](PF 6 ) 2 ·3DMF: C 42.55, H 3.84, N 17.79, Cl 4.74. Found: C 42.92, H 3.49, N 17.92, Cl 5.21. Preparation of [Cu 2 ( m -xpt) 2 ](PF 6 ) 2 (3) To a stirred solution of 1 (200 mg, 0.14 mmol) or 2 (178 mg, 0.14 mmol) in DMF (20 ml), sodium ascorbate (41 mg, 0.21 mmol) was added under N 2 . After 1 h, the yellow solution was slowly diffused with diethyl ether under N 2 for 2 days. The solid was collected by filtration, washed with diethyl ether, and dried to give 3 (164 mg, 85% from 1 ; 156 mg, 81% from 2 ). 1 H NMR (dimethylsulphoxide-d6, DMSO-d 6 , 400 MHz): 5.79 (s, 8H, CH 2 ), 7.43–7.49 (m, 12H, Ar), 8.12 (br, 8H, Ar), 8.43 (br, 4H, Ar), 9.23 (br, 4H, triazole). 13 C NMR (DMSO-d 6 , 125 MHz): 54.3, 122.1, 125.1, 125.9, 128.8, 129.3, 130.1, 136.0, 139.3, 146.0, 147.1, 149.5. ESI-MS: 1059.171 [Cu 2 ( m -xpt) 2 (PF 6 )] + (calcd 1059.154). Anal. Calcd for [Cu 2 ( m -xpt) 2 ](PF 6 ) 2 : C 43.82, H 3.01, N 18.58. Found: C 43.58, H 3.16, N 17.92. Like 1 , this compound also gave microanalyses that were low in N. Addition of a small amount of ether to the formula gives somewhat better agreement; however, there were no signals attributable to ether or to other impurities in the compound’s NMR spectrum. Preparation of [Cu 2 ( m -xpt) 2 ( μ -C 2 O 4 )](PF 6 ) 2 (4) A stirred solution of 1 (200 mg, 0.14 mmol) or 2 (178 mg, 0.14 mmol) in DMF (20 ml) was reduced to [Cu 2 ( m -xpt) 2 ](PF 6 ) 2 ( 3 ) by the addition of sodium ascorbate (41 mg, 0.21 mmol) under N 2 for ~1 h. The resulting yellow solution was exposed to air for reaction with atmospheric CO 2 and slow evaporation of the solvent. After 4–5 days, green octahedron shaped crystals of 4 (see Supplementary Fig. 8a ) had formed when complex 1 was used as starting material. When complex 2 was used as starting material, both green and blue-green crystals (see Supplementary Fig. 8b ) were obtained. Both types of crystals were characterized by X-ray crystallography. The green crystals were found to be the oxalate-bridged dimer 4 ( Fig. 4 and Supplementary Data 3 ), and the blue-green crystalline product was the starting Cu(II) dimer, [Cu 2 ( m -xpt) 2 Cl 2 ](PF 6 ) 2 . The mixture was washed with acetonitrile, which dissolved the blue-green crystals, and 4 (194 mg, 96% from 1 ; 138 mg, 69% from 2 ) was collected by filtration. FTIR (cm −1 ): 1670(s), 1645 (s), 1610 (s), 1454 (s), 839 (vs), 785 (vs), 715 (vs). Anal. Calcd for [Cu 2 ( m -xpt) 2 ( μ -C 2 O 4 )(PF 6 ) 2 ]·2DMF: C 43.37, H 3.50, N 17.51. Found: C 43.48, H 3.52, N 17.58. Preparation of [Cu 2 ( m -xpt) 2 ( μ - 13 C 2 O 4 )](PF 6 ) 2 We synthesized the Cu(I) complex 3 starting from complex 1 under N 2 as discussed above. The solution was transferred into a sealed flask connected to a cuvette. The reaction mixture was purged with nitrogen by four alternating cycles of vacuum and nitrogen. The reaction mixture showed no changes in its ultraviolet–visible spectrum for 48 h. At that point, the N 2 was replaced by 13 CO 2 . The yellow solution progressively turned to green over a period of 128 h; during this period, 13 CO 2 was added periodically to maintain the pressure at ~1 atm. After the reaction was complete, the solution was poured into a watch glass and left for crystallization by slow evaporation of DMF. The crystalline solid was washed with acetone. The IR spectrum of the product, and a difference spectrum showing ν 13C =1651, cm −1 , are in Supplementary Fig. 7 . [Cu 2 ( m -xpt) 2 X 2 ](PF 6 ) 2 (X=NO 3 , Cl) as a host for oxalate To a stirred solution of 1 (200 mg, 0.14 mmol) or 2 (178 mg, 0.14 mmol) in acetonitrile (20 ml), tetrabutylammonium oxalate [31] (80 mg, 0.15 mmol) was added. The mixture was stirred for 30 min and then left for crystallization by slow evaporation of the solvent. The product appeared in the form of yellow-green crystals, which were washed with acetonitrile and air-dried to give 4a (178 mg, 87% from 1 ; 147 mg, 72% from 2 ). X-ray analysis showed that these crystals were the acetonitrile solvate of [Cu 2 ( m -xpt) 2 ( μ -C 2 O 4 )](PF 6 ) 2 , 4a (Cu···Cu=5.462(2) Å), which is isostructural with the DMF solvate 4 ; see Supplementary Table 2 for data and refinement parameters, and Supplementary Data 4 . Removal of bound oxalate from [Cu 2 ( m -xpt) 2 ( μ -C 2 O 4 )](PF 6 ) 2 (4) To a stirred suspension of complex 4 (100 mg, 0.08 mmol) in methanol (50 ml), HNO 3 (aq) or HCl(aq) (2 ml of 0.32 M, 0.64 mmol) was added. The solid dissolved, giving a blue solution (HNO 3 ) or a greenish-yellow solution (HCl), but a precipitate formed after stirring for an additional 3 h. The mixture was filtered and the solid redissolved in a mixture of water and DMF (4:1 v/v), and the solution was poured into a watch glass and left for slow evaporation. After 4–5 days, blue (HNO 3 ) or blue-green (HCl) crystalline product had formed, which was collected, washed with ~5 ml methanol and air-dried. X-ray analysis of the products revealed the formation of the empty Cu(II) macrocycles. With HNO 3 , the product was [Cu 2 ( m -xpt) 2 (H 2 O) 2 ](NO 3 ) 4 ·4DMF ( 5 ; 81 mg, 96%; see crystal structure in Fig. 5 and Supplementary Data 5 ). Anal. Calcd for [Cu 2 ( m -xpt) 2 (H 2 O) 2 ](NO 3 ) 4 ·2H 2 O: C 42.76, H 3.59, N 22.66. Found: C 42.38, H 3.55, N 21.86. With HCl, the previously reported [Cu 2 ( m -xpt) 2 Cl 2 ]Cl 2 ·4DMF 1 (92 mg, 94%) formed. The filtrate from the above reaction was evaporated to dryness. The solid was dissolved in water (2 ml), and the solution neutralized with KOH(aq), and extracted with chloroform. The aqueous phase was acidified with HCl(aq) and again evaporated to dryness to give oxalic acid ( 13 C NMR in DMSO-d 6 , 163.2 ppm; FTIR 1668, cm −1 ). The same procedure carried out on [Cu 2 ( m -xpt) 2 ( μ - 13 C 2 O 4 )](PF 6 ) 2 yielded 13 C labelled oxalic acid (H 2 13 C 2 O 4 ; 1644, cm −1 ). How to cite this article : Pokharel, U. R. et al . Reduction of carbon dioxide to oxalate by a binuclear copper complex. Nat. Commun. 5:5883 doi: 10.1038/ncomms6883 (2014). Accession codes: The X-ray crystallographic coordinates for structures reported in this Article have been deposited at the Cambridge Crystallographic Data Centre (CCDC), under deposition numbers CCDC 1000457 ( 1 ), 1000458 ( 2 ), 984468 ( 4 ), 984469 ( 4a ), and 984470 ( 5 ). These data can be obtained free of charge from The Cambridge Crystallographic Data Centre via www.ccdc.cam.ac.uk/data_request/cif .